A multicentre-bonded [ZnI]8cluster with cubic aromaticity Polynuclear zinc clusters [Zn x ] ( x >2) with multicentred Zn–Zn bonds and +1 oxidation state zinc (that is, zinc(I) or Zn I ) are to our knowledge unknown in chemistry. Here we report the polyzinc compounds with an unusual cubic [Zn I 8 (HL) 4 (L) 8 ] 12− (L=tetrazole dianion) cluster core, composed of zinc(I) ions and short Zn–Zn bonds (2.2713(19) Å). The [Zn I 8 ]-bearing compounds possess surprisingly high stability in air and solution. Quantum chemical studies reveal that the eight Zn 4s 1 electrons in the [Zn I 8 ] cluster fully occupy four bonding molecular orbitals and leave four antibonding ones entirely empty, leading to an extensive electron delocalization over the cube and significant stabilization. The bonding pattern of the cube represents a class of aromatic system that we refer to as cubic aromaticity, which follows a 6 n +2 electron counting rule. Our finding extends the aromaticity concept to cubic metallic systems, and enriches Zn–Zn bonding chemistry. Chemical bonding is the cornerstone of the whole chemistry edifice [1] , [2] . Among the various bonding types, metal–metal (M–M) bonding has been one of the most important themes in inorganic chemistry since Cotton et al. [3] proposed the concept of M–M quadruple bonding in the [Re 2 Cl 8 ] 2− ion in 1964. Especially noteworthy in this field are the findings of novel structures and applications of uncommon low oxidation state (LOS) M–M bonded compounds stabilized by sterically bulky ligands. Great progress has been recently witnessed by successful syntheses of compounds with single M I -M I bonds (for example, M=Zn (ref. 4 ), In (ref. 5 ), Mg (ref. 6 ), Co (ref. 7 ), Cd (ref. 8 )) and those with quintuple M–M bonds between Cr I (ref. 9 ) or Mo I (ref. 10 ). Among those, the landmark discovery of decamethyldizincocene [Cp*ZnZnCp*] (Cp*=C 5 Me 5 ) with a covalent Zn I –Zn I bond by Carmona and coworkers in 2004 initiated the epoch of Zn–Zn bonding chemistry [11] , [12] , [13] , [14] , [15] , [16] , [17] , [18] , [19] , [20] , [21] , [22] , [23] . However, these studies focus on the [Zn I 2 ] 2+ dimeric species that are not sufficiently stable in air [11] . So far, no polyzinc cluster [Zn x ] x + ( x >2) with multicentred Zn I –Zn I bonds are known. Here we report the synthesis, characterization and theoretical analysis of two Zn I compounds with a rare cubic [Zn I 8 (HL) 4 (L) 8 ] 12− (L=tetrazole dianion) cluster containing multicentred Zn–Zn bonds. These Zn I 8 -bearing compounds are surprisingly stable in solutions and in air at temperature far above ambient temperature. Quantum chemical studies reveal extensive electron delocalization over the Zn I 8 cube. Our finding extends the aromaticity concept from the all-metal aromaticity [24] , [25] , [26] , [27] , [28] , [29] , [30] and spherical aromaticity obeying 2( n +1) 2 rule [31] to cubic metal systems. Syntheses To form LOS Zn–Zn-bonded compounds, we designed a series of reactions for the in situ reduction of Zn II compounds under a solvothermal condition. The same approach was used previously for in situ reduction of Cu II and Fe III to yield LOS ions [32] . Here we report the syntheses of two compounds, Na 2.6 K 1.4 {[Na(DMF)] 8 [Zn I 8 (HL) 4 (L) 8 ]}·8H 2 O·2H 2 L·DMF ( 1 ) and Na 3 K 2.33 {K 4 [Na(DMF) 3 ] 1.33 [Zn II Br] 1.33 [Zn I 8 (HL) 4 (L) 8 ]}·2H 2 O·2H 2 L·4DMF ( 2 ) (DMF= N , N '-dimethylformamide), by in situ reactions of K[C(CN) 3 ], NaN 3 and Zn II salts under solvothermal conditions, with the yield of ~26 and ~15%, respectively. 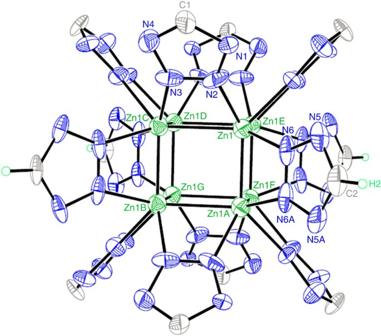Figure 1: Structure of cluster {Zn8(HL)4(L)8}12−in1. Selected bond distances (Å): Zn1–Zn1A (Zn1B–Zn1C, Zn1D–Zn1G, Zn1E–Zn1F)=2.292(2), Zn1–Zn1C (Zn1–Zn1E, Zn1A–Zn1B, Zn1A–Zn1F, Zn1B–Zn1G, Zn1C–Zn1D, Zn1D–Zn1E, Zn1F–Zn1G)=2.4810(18). Thermal ellipsoids are set at the 25% probability level. The crystals of 1 can also be produced by using ZnO or other organonitriles, such as 7,7,8,8-tetracyanoquinodimethane, biphenyl-4,4-dicarbonitrile, 1,1,3,3-tetrakis-cyanopropane and so on, although the yields are much lower and the qualities of the crystals are relatively poor ( Supplementary Table 1 ). Analyses of stability Both 1 and 2 are stable in air, as revealed by powder X-ray diffraction of the samples exposed to air for at least half a year ( Supplementary Figs 1 and 2 ) and thermogravimetry analyses ( Supplementary Fig. 3 ). These two kinds of compounds are insoluble in common organic solvents. However, 1 can easily dissolve in water and recrystallize on adding DMF into water, as is supported by crystal structure analyses of the recrystallized samples. It follows that the [Zn I 8 (HL) 4 (L) 8 ] 12− cluster can stably exist in water, which is further confirmed by the high-resolution electrospray ionization mass spectrometry (ESI-MS) of 1 in water. Series of zinc isotope peaks centred at m/z =738.8141 are clearly observed ( Supplementary Figs 4 and 5 ), and the simulated MS patterns of the molecular fragment {[Zn 8 (HL) 4 (L) 8 ][Na 4 (H 2 O) 2 ]+6H} 2− (calcd. 738.8128) containing [Zn 8 (HL) 4 (L) 8 ] 12− cluster match well with the corresponding experimental isotope peaks. This high stability of the [Zn I 8 (HL) 4 (L) 8 ] 12− cluster is in striking contrast with the existing [Zn I 2 ] 2+ compounds, which survived only in low temperature and were so air sensitive as to burn out spontaneously [4] . Structural analyses The molecular structures of 1 and 2 were determined by single-crystal X-ray diffraction, and their non-hydrogen atoms were also identified by X-ray photoelectron spectroscopy (XPS) analyses ( Supplementary Fig. 6 ). In addition, small molecules or cations within the pores of 1 and 2 , such as DMF, Na + , K + , H 2 L and H 2 O, were characterized by 1 H and 13 C nuclear magnetic resonance (NMR), ion chromatography ( Supplementary Fig. 7 ), infrared spectra (IR), elemental analyses and inductively coupled plasma (ICP). While crystallized in different space groups of I 4/ m for 1 and P -43 m for 2 , they possess a unique tetragonally distorted Zn I 8 cubic cluster with direct multicentred Zn–Zn bonding, and the Zn I 8 core is supported by twelve tetrazole rings, forming [Zn I 8 (HL) 4 (L) 8 ] 12− motifs. In addition to the Zn–Zn bonds, the adjacent two Zn I ions are further connected by two N atoms from the tetrazole ring ligands, which orient along the corresponding twelve edges of the Zn I 8 cube. Thus, each Zn I ion coordinates to three N atoms of the tetrazole ligands and three neighbouring Zn I ions in the cube. Different from all previously reported [Zn I 2 ] 2+ species [11] , where various bulky ligands, for example, C 5 Me 5 , [{(2,6-i-Pr 2 C 6 H 3 )N(Me)C} 2 CH], and [2,6-(2,6-i-Pr 2 C 6 H 3 )C 6 H 3 ], were utilized to protect the Zn I –Zn I bond, compounds 1 and 2 provide the first example of stable Zn I –Zn I bonds supported only by small tetrazole ligands. In these compounds, eight Zn I ions act as the vertices of the distorted cube, forming Zn I 8 core with D 4h symmetry in 1 and D 2d symmetry in 2 . There are twelve Zn I –Zn I bonds in 1 ( Fig. 1 ), with four Zn I –Zn I bond lengths of 2.292(2) Å and eight Zn I –Zn I ones of 2.4810(18) Å. All these twelve Zn I –Zn I bond lengths are smaller than the sum of Pauling’s single-bond metallic radii (2.50 Å) (ref. 2 ), suggesting the existence of direct Zn–Zn bonds. In the Zn I 8 cube of 2 ( Fig. 2 ), due to the lower local symmetry, twelve Zn I –Zn I bonds divide into three groups, corresponding to three types of bond lengths of 2.394(2), 2.766(2) and 2.2713(19) Å, where the latter is slightly shorter than the shortest Zn–Zn bonds (2.295 Å) in Zn 2 (ŋ 5 -C 5 Me 4 Et) 2 (ref. 14 ), and the four Zn I –Zn I bonds of 2.766(2) Å are weaker. Figure 1: Structure of cluster {Zn 8 (HL) 4 (L) 8 } 12− in 1 . Selected bond distances (Å): Zn1–Zn1A (Zn1B–Zn1C, Zn1D–Zn1G, Zn1E–Zn1F)=2.292(2), Zn1–Zn1C (Zn1–Zn1E, Zn1A–Zn1B, Zn1A–Zn1F, Zn1B–Zn1G, Zn1C–Zn1D, Zn1D–Zn1E, Zn1F–Zn1G)=2.4810(18). Thermal ellipsoids are set at the 25% probability level. 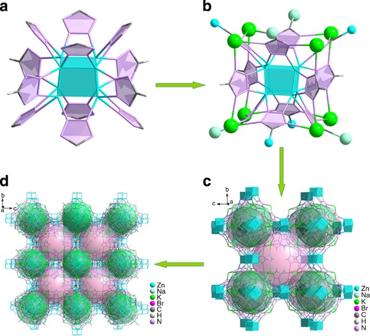Figure 2: Three-dimensional (3D) framework structure of2. (a) The {Zn8(HL)4(L)8}12−cluster and ZnI8cube structure (blue cube) in2. (b) The connections among the cluster and Na+, K+, ZnII. (c) Eight clusters as nearest neighbours around each cluster. (d) The 3D framework with the alternatively arranged closed cages (green) and open cages (pink). Full size image Figure 2: Three-dimensional (3D) framework structure of 2 . ( a ) The {Zn 8 (HL) 4 (L) 8 } 12− cluster and Zn I 8 cube structure (blue cube) in 2 . ( b ) The connections among the cluster and Na + , K + , Zn II . ( c ) Eight clusters as nearest neighbours around each cluster. ( d ) The 3D framework with the alternatively arranged closed cages (green) and open cages (pink). Full size image In 1 , each [Zn I 8 (HL) 4 (L) 8 ] 12− cluster is linked to eight such clusters as its nearest neighbours by sixteen Na + ions, forming a three-dimensional metal-organic framework ( Supplementary Figs 8 and 9 ). In 2 , the C and N atoms in the [Zn I 8 (HL) 4 (L) 8 ] 12− cluster coordinate to external Zn II , Na + and K + ions, generating two types of cages ( Supplementary Fig. 10 ). The small closed cages and large open cages are alternately arranged, giving a fascinating three-dimensional framework ( Fig. 2 ). Each closed cage consists of six [Zn I 8 (HL) 4 (L) 8 ] 12− clusters, four Zn II , four Na + and twelve K + , while each open cage is constructed by twelve [Zn I 8 (HL) 4 (L) 8 ] 12− clusters, four Zn II , four Na + and twenty-four K + . These different types of ions connected with the [Zn I 8 (HL) 4 (L) 8 ] 12− cluster significantly influence the ultraviolet–visible and luminescence spectra of 1 and 2 ( Supplementary Fig. 11 ). Spectrocopic and theoretical studies The existence of Zn I –Zn I bonds in 1 and 2 is supported by both experimental and theoretical evidences. From the measured Raman spectra of 1 and 2 ( Supplementary Fig. 12 ), several low-frequency vibration peaks involving the contribution of Zn–Zn stretching modes are observed between 100 and 400 cm −1 (refs 18 , 19 , 20 ), but a clear-cut assignment is difficult due to significant Zn–Zn and Zn–L modes mixing. Geometry optimizations, bond order and electron localization function (ELF) calculations using density functional theory methods also confirm direct Zn–Zn bond. We find that the different Zn–Zn distances in 1 and 2 are related to the varied donation ability of the tetrazole ligand with different outside cations, indicating the tetrazole ligands also play a role in stabilizing the Zn I 8 clusters. The theoretically predicted Zn–Zn distances are 2.43, 2.46 Å in 1 , and 2.32, 2.42 and 2.81 Å in 2 ( Supplementary Table 2 ), which agree well with their corresponding experimental values of 2.29, 2.48 Å in 1 and 2.27, 2.39 and 2.77 Å in 2 . The Mayer bond orders of Zn–Zn bonds are calculated as 0.32 and 0.35 in 1 , as well as 0.48, 0.34, and 0.14 in 2 , consistent with each Zn connecting to three adjacent Zn in the cube. The ELF contours also show significant electron-pair density along the Zn–Zn bond, supporting direct Zn–Zn bonding in the clusters ( Fig. 3 ). 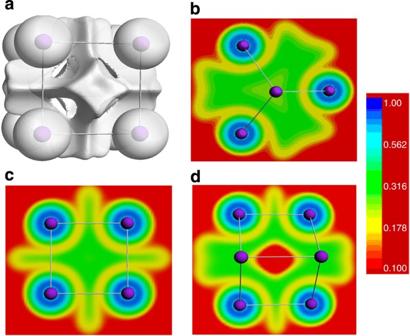Figure 3: ELFs for Zn88+. (a) The isosurface of the cube. (b) The triangular surface. (c) The square surface. (d) The diagonal rectangular surface. Figure 3: ELFs for Zn 8 8+ . ( a ) The isosurface of the cube. ( b ) The triangular surface. ( c ) The square surface. ( d ) The diagonal rectangular surface. Full size image As Zn I is usually much less stable than Zn II in chemistry, it is remarkable that all the zinc atoms in the Zn 8 core of 1 and 2 exist in a +1 oxidation state. The XPS data reveal that the binding energy of Zn ions appears at 1019.5 eV for 1 and 1020.1 eV for 2 ( Supplementary Fig. 6 ), which is markedly smaller than the reported Zn 2p 3/2 binding energy (1021.8 eV) of Zn II ions [33] . As LOS always has smaller binding energy than its higher one, the large deviation to our experimental values from those of Zn II ions suggests the presence of LOS Zn ions in 1 and 2 . By comparison with 1 , the Zn II ions coordinated to Br atoms in 2 cause the broadening and blue-shift of the XPS peaks, thus accounting for their difference. We also carried out density functional theory calculations on the model clusters [Na 8 Zn 8 (HL) 4 (NaL) 8 ] n+ by assuming Zn I ( n =4) or Zn II ( n =12). The geometry optimized for the [Zn I 8 ] cluster agrees well with the experimental crystal structure, whereas that of [Zn II 8 ] will lead to extremely long Zn…Zn distance and eventually the collapse of [Zn II 8 ] cluster, providing additional credence for Zn I in 1 and 2 . X-ray absorption near-edge structures We further performed X-ray absorption near-edge structure (XANES) analyses of four samples, including 1 and 2 together with Zn(NO 3 ) 2 ·6H 2 O and Zn foil as standard control groups ( Fig. 4 ). Although no previous XANES data of Zn I ions are reported, there exists a linear correlation between the Zn K-edge energies of these samples and their formal oxidation states. Our XANES data show that the Zn K-edge energies in 1 and 2 exactly correspond to the +1 oxidation state, thus providing an unequivocal evidence for the existence of Zn I ions in these compounds, originated from the reduction of Zn II ions caused by the cleavage of C–C bonds. 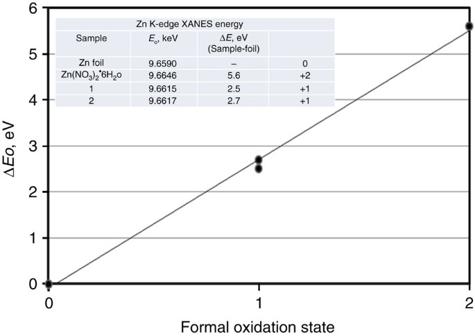Figure 4: The change of Zn K-edge energy versus oxidation state. The Zn foil edge energy (9.6590, keV) is selected as the reference energy, that is, ΔEo=0. Inset: the Zn K-edge XANES energy. Figure 4: The change of Zn K-edge energy versus oxidation state. The Zn foil edge energy (9.6590, keV) is selected as the reference energy, that is, Δ E o =0. Inset: the Zn K-edge XANES energy. Full size image To elucidate the bonding of the Zn I 8 cube and the special thermal stability of [Zn I 8 (HL) 4 (L) 8 ] 12− motifs in 1 and 2 , we have further investigated the Zn–Zn bonding properties and electronic structures of the [Zn I 8 ] systems using selected O h , D 4h and D 2d model clusters. Our results show that the clusters have closed-shell electron configuration ( Fig. 5 ), consistent with the EPR-silence and diamagnetic feature of the samples ( Supplementary Figs 13 and 14 ). Inasmuch as Zn I ion only possesses one 4 s electron, eight delocalized molecular orbitals (MOs) of the Zn I 8 cube are formed through overlap of the 4 s orbitals, with slight mixing from the Zn 4 p and Zn 3 d orbitals. Among them, four bonding orbitals with a 1g and t 1u symmetry are fully occupied, giving a ground-state electronic configuration of (a 1g ) 2 (t 1u ) 6 , whereas four antibonding orbitals with t 2g and a 2u symmetry are completely empty. The bonding pattern of the eight MOs is comparable to those of Au 3 + and benzene molecules that have the famous planar σ- and π-aromaticity [34] and obey Hückel’s 4 n +2 rule ( Supplementary Fig. 15 ). This bonding pattern represents a rare type of aromaticity, which we refer to as cubic aromaticity. Such systems follow a 6 n +2 electron counting rule or approximately the 2( n +1) 2 rule [29] , which might help to search for heteroatomic cubic clusters with apt number of electrons. 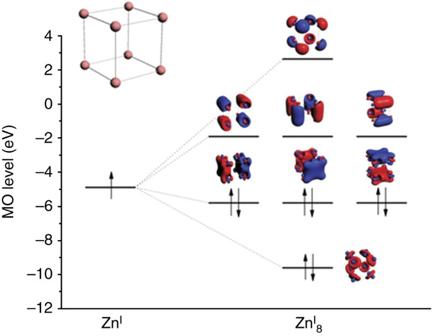Figure 5: The bonding pattern in ZnI8with cubic aromaticity. Levels of ZnI8are shifted relative to ZnI. Figure 5: The bonding pattern in Zn I 8 with cubic aromaticity. Levels of Zn I 8 are shifted relative to Zn I . Full size image This special cubic aromaticity arises from the electron delocalization over the entire Zn I 8 cube. The calculated nucleus-independent chemical shift indices at the cubic-, face-, bond-centre display considerable negative values, which are comparable to those in benzene, also confirming the special aromaticity of the Zn I 8 cube ( Supplementary Table 3 ). Through theoretical analyses of the Zn I 8 cube using analytic Hückel MO model and Kohn–Sham MOs, the estimated resonance energy (4.00 β ZnZn ) appears to be comparable with that of benzene (2.00 β CC ), far larger than 1.00 β ZnZn in reported Zn I 2 compounds with Zn–Zn bonds, where β is the resonance integral. Furthermore, the additional multi-centre bonding among the eight Zn atoms provides extra stabilization than the two-centre two-electron bonding in Zn 2 compounds. As a result, the cubic aromaticity, additional Zn 4p orbital interactions, and the strong metal-ligand interactions are responsible for the robustness of the [Zn I 8 ] core and the unique stability of the octanuclear Zn I compounds. Our finding of the stable [Zn I 8 ] motif to form self-assembled materials may have practical applications. Particularly, as these materials with specially stabilized Zn I and the high energy density tetrazole rings [35] can undergo explosive combustion above 300 °C, they might find applications as propellants and high temperature explosives. The stable [Zn I 8 ] core with electron delocalization might be used to construct robust non-linear optical materials. Insofar as the special stability of the Zn I 8 cube, we anticipate that the cubic aromaticity via s -, p -, d -, f -type atomic orbital overlap might also exist in other cubic metal cluster materials. Synthesis of 1 Compound 1 can be obtained by the following five methods A–E, among which method A has the highest yield. Caution: owing to the explosive potential of NaN 3 and tetrazole-based compounds, only a small amount of material should be used and handled with care! Method A The mixture of Zn(ClO 4 ) 2 ·6H 2 O (74.5 mg, 0.2 mmol), NaN 3 (65 mg, 1.0 mmol), NH 4 F (11.1 mg, 0.3 mmol) and K[C(CN) 3 ] (12.9 mg, 0.1 mmol) in DMF (6 ml) was sealed in a 25-ml Teflon-lined stainless steel autoclave and heated at 155 °C for 4 days and then cooled to room temperature at the rate of 1 °C per hour. Finally, colourless octahedral crystals of 1 were obtained directly, then washed with DMF and dried in air. Yield: 15.5 mg, 26% based on K[C(CN) 3 ] (0.1 mmol). ICP analysis: Zn/Na/K molar ratio of 1:1.5:0.18. Anal. Calcd. (%) for C 41 H 87 N 65 O 17 K 1.4 Na 10.6 Zn 8 : C, 19.06; H, 3.39; N, 35.23. Found: C, 19.45; H, 4.12; N, 35.76. Selected IR (KBr, cm –1 ): 3,426(vs), 2,934(w), 1,659(vs), 1,434(s), 1,390(s), 1,148(s), 1,106(m), 1,064(s), 950 (s), 771(w). High-resolution ESI-MS for 1 in H 2 O/CH 3 OH was performed and analysed with the anion mode. 1 H NMR (400 MHz; D 2 O) δ 7.70 (1H), 2.59 (3H), 2.58 (3H); 13 C NMR (400 MHz; D 2 O) δ 165.9, 164.8, 67.9, 36.5 31.2. As is usual, the absence of some H signals in tetrazole 1 H NMR spectra is due to the fast proton exchange. Remarkably, the colourless polyhedral crystals ( 1a ) were isolated after recrystallization of 1 from a H 2 O/DMF mixture at room temperature, which were determined by single-crystal structure analysis. This result indicates that the [Zn I 8 (HL) 4 (L) 8 ] 12− cluster remains intact in solvent because Zn I ions in water is very unstable and easily disproportionates into Zn(0) and Zn II . 1a would not be obtained by recrystallization if [Zn I 8 (HL) 4 (L) 8 ] 12− cluster had undergone the disproportionation reaction to decompose. Unfortunately, effort of exchanging free Na + and K + in 1 by other cations such as NH 4 + , [N(CH 3 ) 4 ] + , and [N(C 2 H 5 ) 4 ] + was not successful. Method B A mixture of ZnO (24.4 mg, 0.3 mmol), NaN 3 (19.5 mg, 0.3 mmol) and K[C(CN) 3 ] (12.9 mg, 0.1 mmol) in DMF (6 ml) was sealed in a 25-ml Teflon-lined stainless steel autoclave and heated at 160 °C for 4 days and then cooled to room temperature at a rate of 1 °C per hour to form colourless octahedral crystals ( 1b ), but with low yield. Method C A mixture of ZnBr 2 (45.0 mg, 0.2 mmol), NaN 3 (39 mg, 0.6 mmol) and 1,1,3,3-tetrakis-cyanopropane (14.4 mg, 0.1 mmol) in DMF (6 ml) was sealed in a 25-ml Teflon-lined stainless steel autoclave and heated at 160 °C for 4 days and then cooled to room temperature at the rate of 1 °C per hour. Finally, colourless square-pyramidal crystals ( 1c ) were obtained directly, but with poor quality and low yield. Method D A mixture of ZnBr 2 (45.0 mg, 0.2 mmol), NaN 3 (39 mg, 0.6 mmol) and 7,7,8,8-tetracyanoquinodimethane (20.4 mg, 0.1 mmol) in DMF (6 ml) was sealed in a 25-ml Teflon-lined stainless steel autoclave and heated at 160 °C for 4 days and then slowly cooled to room temperature at the rate of 1 °C per hour. Finally, colourless square-pyramidal crystals ( 1d ) were obtained directly, but with poor quality and low yield. Method E A mixture of ZnBr 2 (67.6 mg, 0.3 mmol), NaN 3 (39 mg, 0.6 mmol) and biphenyl-4,4′-dicarbonitrile (10.2 mg, 0.05 mmol) in DMF (6 ml) was sealed in a 25-ml Teflon-lined stainless steel autoclave and heated at 160 °C for 4 days and then slowly cooled to room temperature at the rate of 1 °C per hour. Finally, colourless square-pyramidal crystals ( 1e ) were obtained directly, but with poor quality and low yield as well. Synthesis of 2 The mixture of ZnBr 2 (135.2 mg, 0.6 mmol), NaN 3 (39 mg, 0.6 mmol) and K[C(CN) 3 ] (25.8 mg, 0.2 mmol) in DMF (6 ml) was sealed in a 25-ml Teflon-lined stainless steel autoclave and heated at 170 °C for 4 days and then slowly cooled to room temperature at the rate of 1 °C per hour. Finally, pale-yellow cubic crystals of 2 were obtained directly and were then washed with ethanol and dried in air. Yield: 22.5 mg, 15% based on K[C(CN) 3 ] (0.2 mmol). ICP analysis: Zn/Na/K molar ratio of 1:0.44:0.6. Anal. Calcd. (%) for C 38 H 68 N 64 O 10 Br 1.33 Na 4.33 K 6.33 Zn 9.33 : C, 17.26; H, 2.59; N, 33.89. Found: C, 17.61; H, 2.33; N, 34.11. Selected IR (KBr, cm −1 ): 3,440(vs), 2,932(w), 1,663(vs), 1,434(s), 1,390(s), 1,255(w), 1,144(s), 1,101(m), 1,069(s), 952 (s), 772(w). 1 H NMR (400 MHz; D 2 O) δ 7.75 (1H), 2.79 (3H), 2.67 (3H); 13 C NMR (400 MHz; D 2 O) δ 165.9, 164.9, 67.8, 36.8, 31.3. X-ray crystallographic analyses Data were collected on an Oxford SuperNova (TM) CCD Diffractometer with a SuperNova X-ray Source (Mo-Kα). The structure was solved using SHELXS-97 and refined using SHELXL-97 contained in Olex2 programme. All hydrogen atoms were attached to their parent atom in a riding model, using the appropriate command. See Supplementary Data 1 and 2 for the CIF crystallographic information file, and Supplementary Methods for the discussion of data collection and refinement. Characterization methods Both compounds were characterized using a wide range of spectroscopy and other experimental techniques (such as powder X-ray diffraction, thermogravimetry analyses, ESI-MS, ICP, XPS, EPR, XANES). Details are provided. See Supplementary Methods for Material characterization. Theoretical details The theoretical analyses were performed to investigate the local symmetry of the cluster, the optimal spin multiplicity, oxidation state of Zn, effects of external R (Na, H, F and BrZn) ions on the structure of [Zn 8 (RL) 12 ] 4− , MO analysis and nucleus-independent chemical shift indices, NBO and ELF analysis of the direct Zn–Zn bonding (see Supplementary Methods ). Accession codes: The X-ray crystallographic coordinates for structures reported in this Article have been deposited at the Cambridge Crystallographic Data Centre (CCDC), under deposition number CCDC 879470 for 1 and 879472 for 2 . These data can be obtained free of charge from The Cambridge Crystallographic Data Centre via www.ccdc.cam.ac.uk/data_request/cif . How to cite this article: Cui, P. et al. A multicentre-bonded [Zn I ] 8 cluster with cubic aromaticity. Nat. Commun. 6:6331 doi: 10.1038/ncomms7331 (2015).